Dendritic cell-mediated survival signals in Eμ-MycB-cell lymphoma depend on the transcription factor C/EBPβ The capacity of dendritic cells (DCs) to regulate tumour-specific adaptive immune responses depends on their proper differentiation and homing status. Whereas DC-associated tumour-promoting functions are linked to T-cell tolerance and formation of an inflammatory milieu, DC-mediated direct effects on tumour growth have remained unexplored. Here we show that deletion of DCs substantially delays progression of Myc-driven lymphomas. Lymphoma-exposed DCs upregulate immunomodulatory cytokines, growth factors and the CCAAT/enhancer-binding protein β (C/EBPβ). Moreover, E μ -Myc lymphomas induce the preferential translation of the LAP/LAP* isoforms of C/EBPβ. C/EBP β −/− DCs are unresponsive to lymphoma-associated cytokine changes and in contrast to wild-type DCs, they are unable to mediate enhanced E μ -Myc lymphoma cell survival. Antigen-specific T-cell proliferation in lymphoma-bearing mice is impaired; however, this immune suppression is reverted by the DC-restricted deletion of C/EBP β. Thus, we show that C/EBPβ-controlled DC functions are critical steps for the creation of a lymphoma growth-promoting and -immunosuppressive niche. Dendritic cells (DCs) act as specialized antigen-presenting cells, and when these cells interact with T cells, they can initiate either immunity or tolerance in the naive T lymphocytes [1] , [2] . Defects in DC maturation can result in non-responsiveness of the immune system to tumours, an effect that is mediated by changes in cytokine and growth factor expression [3] , [4] , [5] , and by an altered expression of costimulatory molecules on the cell surface. However, the molecular mechanisms that provide DCs with a direct tumour-promoting function are incompletely understood. Polarized inflammation predisposes to initiation and promotion of cancer [6] . Mediators of this condition are often myeloid cells releasing pro-inflammatory chemokines and cytokines. Tumour-necrosis factor-α (TNF-α), interleukin (IL)-6, IL-1, IL-17 and IL-23 are among the best characterized pro-inflammatory cytokines in the tumour microenvironment, and depending on the murine organ model investigated they are often associated with a tumour-promoting effect in solid tumours [7] , [8] . Inflammation-modulating chemokines such as CCL2, CCL5, CCL17, CCL22 and CXC-chemokines act indirectly on tumour promotion because they contribute to the recruitment and polarization of macrophages, CD4 + T helper 2 lymphocytes, immature myeloid-derived suppressor cells (MDSCs) and neutrophils as well. The predominating transcription factors controlling the pro-inflammatory status are NF-κB, AP-1, STATs and CCAAT/enhancer-binding protein β (C/EBPβ) [9] . The paradigm for the association between inflammation and tumour pathogenesis has evolved from epithelial tumours [6] , the best characterized examples include cancers of the colon, stomach, breast and prostate, but also for hepatocellular carcinoma an intimate relationship between inflammation and tumorigenesis has been suggested [7] , [8] . It remains unclear, however, whether the conditions for the pathogenesis of lymphoid malignancies are distinct from the conditions in solid tumours and their metastasis. The cancer cell microenvironment has to be shaped from cell types normally absent from the organ-specific niche and involves recruitment of myeloid, lymphoid and endothelial cell types. In lymphoma, malignant lymphocytes home within an environment that is ontogenetically optimized for lymphocyte growth and survival. Gene expression profiling in follicular lymphoma has revealed a non-neoplastic immune response signature type 2, which has been reported to be associated with an inferior survival in patients [10] . Immune response signatures were developed by the separation of sorted CD14 + cells, a CD19 + malignant and a CD19 − nonmalignant subpopulation. This procedure permitted the determination of the cellular origin of survival-associated gene expression patterns in whole-tissue biopsy specimen and reflects the nature of the infiltrating immune cells. The less favourable type 2 signature contains many genes that are preferentially expressed in macrophages and DCs. Further support for the hypothesis that indolent and aggressive lymphoma progression is also determined by the cellular microenvironment, in addition to genomic aberrations of the malignant cells [11] , [12] , is derived from gene expression profiling in diffuse large B-cell lymphomas. It has been shown that survival of these patients is strongly influenced by immune cell infiltration, fibrosis and angiogenesis, collectively grouped as stromal-1 and -2 signatures [13] . However, the functional implications of lymphoma immune cell infiltration on the antitumour immune response in vivo remain unclear. Previously, we showed that the chemokine receptor CCR7 navigates B-lymphoma cells derived from E μ -Myc transgenic mice into a growth-supporting niche in secondary lymphoid organs (SLOs), where the tumour cells lodge adjacent to fibroblastic reticular cells (FRCs) and DCs [14] . We report here that the transcription factor C/EBPβ is upregulated specifically in DCs when mice were challenged with E μ -Myc lymphoma B cells. C/EBPβ-induced transcriptional alterations are required for the induction of pro-inflammatory cytokines and result in lymphoma progression. In addition, lymphoma-bearing mice exhibit a reduced T-cell antigen responsiveness, which is ameliorated by the DC-specific deletion of the transcription factor C/EBP β. Our data establish a lymphoma-promoting function of DCs that is governed by the transcription factor C/EBPβ. Progression of a Myc-driven B-cell lymphoma depends on DCs To study the role of DCs in lymphoma formation, we transferred lymphoma B cells from diseased E μ -Myc mice intravenously (i.v.) into congenic recipients. In contrast to tumours derived from transgenic E μ -Myc mice, transplantation of lymphoma B cells allows for a better synchronization of disease progression and localization; in particular, this approach has proven suitable for dissecting early growth-promoting conditions [14] . Lymphoma cells (CD45.2 + ) were found predominantly in the T-cell zone of the white pulp in the spleen, where they tightly intermingled with FRCs (gp38 + ) and DCs (CD11c + ; Fig. 1a ). 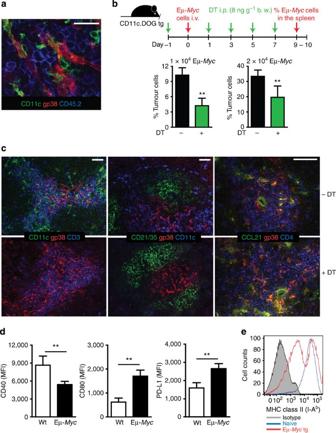Figure 1: DCs enhanceEμ-Myclymphoma progressionin vivo. (a) B6 mice (CD45.1+) were transplanted i.v. with congenic 1 × 105Eμ-Myclymphoma cells. Tumour cells (CD45.2+), gp38+FRC network and DCs (CD11c+) are shown with confocal microscopy (representative z-stack, scale bar, 25 μm) 9–11 days after transfer. Photograph is representative of three independent experiments,n=4–5 mice per experiment. (b)CD11c.DOGmice were treated repeatedly with DT i.p. (Supplementary Fig. 1a). Mice were challenged with 1 × 104or 2 × 104Eμ-MycGFP cells i.v. Tumour load in spleens of DC-depleted mice (green bars,n=3, left panel;n=9, right panel) compared with controls (black bars,n=3, left panel;n=5, right panel) was assessed using GFP-expression in flow cytometry at days 9–10 (n=3 independent experiments). (c)CD11c.DOGmice were transplanted with 1 × 105Eμ-Myclymphoma cells and further treated as inb. Spleen sections were stained after 10 days for the expression of stromal subpopulations with the markers gp38, CD11c and CD21/CD35 (FDC); CD3 and CD4 delineate the T-cell zone. Spleen sections from DT-treated and -untreated mice were also co-stained for CD4, gp38 and CCL21, shown are merged images;n=2–3 mice per group. Scale bars, 50 μm. (d) Expression of costimulatory molecules on CD11c+-gated viable cells from Wt (n=4–7) and Eμ-Myctransgenic mice (3–5 months,n=6-7). Values are expressed as the mean fluorescence intensities (MFIs), and graphs depict means±s.e.m.; inba Student’st-test was applied; indthe Mann–Whitney test was used. *P<0.05; **P<0.01. (e) MHC class II expression on CD11c+DCs in Wt (n=4–7) and Eμ-Myctransgenic mice (3–5 months,n=6–7). One representative histogram is shown. Figure 1: DCs enhance E μ -Myc lymphoma progression in vivo . ( a ) B6 mice (CD45.1 + ) were transplanted i.v. with congenic 1 × 10 5 Eμ-Myc lymphoma cells. Tumour cells (CD45.2 + ), gp38 + FRC network and DCs (CD11c + ) are shown with confocal microscopy (representative z-stack, scale bar, 25 μm) 9–11 days after transfer. Photograph is representative of three independent experiments, n =4–5 mice per experiment. ( b ) CD11c.DOG mice were treated repeatedly with DT i.p. ( Supplementary Fig. 1a ). Mice were challenged with 1 × 10 4 or 2 × 10 4 Eμ-Myc GFP cells i.v. Tumour load in spleens of DC-depleted mice (green bars, n =3, left panel; n =9, right panel) compared with controls (black bars, n =3, left panel; n =5, right panel) was assessed using GFP-expression in flow cytometry at days 9–10 ( n =3 independent experiments). ( c ) CD11c.DOG mice were transplanted with 1 × 10 5 Eμ-Myc lymphoma cells and further treated as in b . Spleen sections were stained after 10 days for the expression of stromal subpopulations with the markers gp38, CD11c and CD21/CD35 (FDC); CD3 and CD4 delineate the T-cell zone. Spleen sections from DT-treated and -untreated mice were also co-stained for CD4, gp38 and CCL21, shown are merged images; n =2–3 mice per group. Scale bars, 50 μm. ( d ) Expression of costimulatory molecules on CD11c + -gated viable cells from Wt ( n =4–7) and Eμ- Myc transgenic mice (3–5 months, n =6-7). Values are expressed as the mean fluorescence intensities (MFIs), and graphs depict means±s.e.m. ; in b a Student’s t -test was applied; in d the Mann–Whitney test was used. * P <0.05; ** P <0.01. ( e ) MHC class II expression on CD11c + DCs in Wt ( n =4–7) and Eμ- Myc transgenic mice (3–5 months, n =6–7). One representative histogram is shown. Full size image Previously, we showed that FRCs support the survival of Eμ- Myc lymphoma cells in vitro and in vivo [14] ; however, the functional contribution of DCs in this B-cell lymphoma model remained elusive. To define the functional consequences of the DC–Eμ- Myc lymphoma cell interaction, we employed the CD11c.DOG mouse strain ( Supplementary Fig. 1a ), which allows for the temporary selective ablation of DCs through the administration of diphtheria toxin (DT). CD11c + -DC depletion in lymphoma-challenged mice significantly retarded lymphoma progression in the spleen, indicating that DCs might have a direct tumour-promoting function ( Fig. 1b ). Despite the strong reduction of DCs in CD11c.DOG mice (+DT), other stroma cell populations within the spleen remained unaffected. The gp38 + FRC network maintained the provision of the chemokine CCL21, as evidenced by gp38 + CCL21 + costaining ( Fig. 1c ). Likewise, the B-cell zone staining of CD21 + CD35 + follicular DCs showed an intact network. We conclude that depletion of DCs still allows for a CCR7-dependent recruitment of E μ -Myc lymphoma B cells, as facilitated by FRCs. A transgenic ovarian cancer model has exhibited a time-dependent downregulation of major histocompatibility complex (MHC) class II and CD40 expression but higher levels of PD-L1 in DCs derived from advanced tumours (>35 days, macroscopic tumour mass), as compared with DCs from mice challenged for shorter periods (≈7 days) [15] . To examine an advanced tumour condition in lymphoma, we isolated splenic DCs from transgenic diseased Eμ- Myc mice (ages 3–5 months) and determined their costimulatory molecule surface expression. We identified a reduction in the activating costimulator CD40, no change in CD86 ( Supplementary Fig. 1c ), but higher levels of CD80 and a higher expression of the T-cell-inhibitory costimulatory molecule PD-L1 compared with DCs (CD11c +high MHC class II +high ) in tumour-naive mice ( Fig. 1d , Supplementary Fig. 1b ). In addition, we observed a downregulation of MHC class II molecules in tumour-exposed DCs in a CD11c + subset, visible as a double-peak distribution in a histogram or as two distinguishable subpopulations in contour plots ( Fig. 1e , Supplementary Fig. 1c ). Together, our data indicate that lymphoma progression is associated with an alteration in DC phenotypes, leading to opposing changes in the expression of activating versus inhibitory maturation markers, and that, functionally, DCs support lymphoma growth in vivo . Transfer of E μ -Myc lymphoma B cells alters DC subsets Tumour-induced immune suppression is associated with the expression of the transcription factor C/EBPβ in the context of MDSCs [16] . Cytokines produced by various experimental tumours including granulocyte–macrophage colony-stimulating factor (GM-CSF) and IL-6 allow for a profound alteration in myelopoiesis regulation, in this process C/EBPβ could serve as a signalling target. Hence, we asked whether C/EBPβ could also influence DC differentiation and function in context of a Myc-driven B-cell lymphoma. We assessed whether E μ -Myc lymphoma cell homing to splenic white pulp influences DC differentiation and activation, comparing splenic CD11c + DCs from tumour-naive and tumour-challenged mice ( Fig. 2 , Supplementary Fig. 2 ). In wild-type (Wt, B6) E μ -Myc lymphoma cell recipients, we identified a moderate decrease in the CD11c + CD4 + population and an increase in the CD11c + double-negative (DN; CD4 − CD8 − ) population, which produces the highest amounts of interferon (IFN)-γ [1] . Wt DCs derived from transplanted tumours maintained comparable levels of MHC class II (I-A b ) and the costimulatory molecule CD80, whereas CD86 was modestly upregulated. Within the resident CD11c + CD8 + DC subpopulation, we found a reduction in the CD205 + subset in lymphoma-bearing mice. CD205 functions as a receptor for CpG oligodeoxynucleotides, and its deficiency leads to impaired DC maturation [17] , [18] . Thus, a fraction of tumour-resident DCs might be compromised in their capacity to capture antigens. 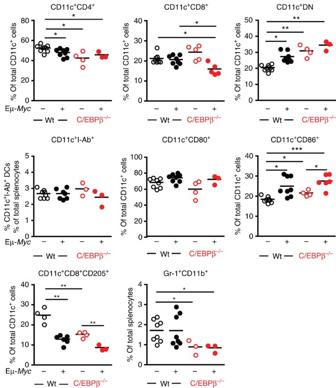Figure 2: DC subset composition is influenced byEμ-Myclymphoma. Splenic DC subsets from naive (n=4–8), WtEμ-Myc-transplanted mice (d 10–13,n=6–8), naiveCD11c.Cre × C/EBPβflox/flox(C/EBPβ−/−;n=3–5) andEμ-Myc-transplantedC/EBPβ−/−mice (n=3–6) were analysed with flow cytometry (Wt,n=3 andC/EBPβ−/−,n=2 independent experiments). CD11c+cells (dot blot; seeSupplementary Fig. 2) were gated, the gate applied to secondary marker expression, and percentages of double- or triple-stained DC subsets depicted. A Mann–Whitney test was applied; *P<0.05; **P<0.01; ***P<0.001. Figure 2: DC subset composition is influenced by E μ -Myc lymphoma. Splenic DC subsets from naive ( n =4–8), Wt Eμ-Myc -transplanted mice (d 10–13, n =6–8), naive CD11c.Cre × C/EBP β flox/flox (C/EBPβ −/− ; n =3–5) and Eμ-Myc -transplanted C/EBP β −/− mice ( n =3–6) were analysed with flow cytometry (Wt, n =3 and C/EBP β −/− , n =2 independent experiments). CD11c + cells (dot blot; see Supplementary Fig. 2 ) were gated, the gate applied to secondary marker expression, and percentages of double- or triple-stained DC subsets depicted. A Mann–Whitney test was applied; * P <0.05; ** P <0.01; *** P <0.001. Full size image To explore the function of C/EBPβ, we generated CD11c.Cre × C/EBP β flox/flox mice in which a selective deletion of C/EBP β in DCs (also referred to as C/EBP β −/− ) was achieved. Most striking differences between Wt and C/EBP β −/− DCs were seen in the CD11c + DN subset; the frequencies among all CD11c + DCs were ≈10% higher in C/EBP β −/− DCs, even without tumour challenge ( Fig. 2 ). Conversely, deletion of C/EBP β was associated with a reduction in the CD11c + CD8 + CD205 + DC subpopulation. In general, changes in the frequencies between tumour-naive and tumour-exposed DC subsets were similar for individual markers, regardless of the C/EBP β genotype. In contrast to several other tumour models, frequencies of MDSCs (Gr-1 + CD11b + ) were identical between Wt naive and tumour-challenged spleens ( Fig. 2 ) [19] ; MDSC subpopulations were not further differentiated. Loss of C/EBPβ decreased this frequency approximately twofold; however, tumour challenge had no additional effect ( Fig. 2 ). Collectively, we conclude that even a short-term lymphoma challenge can elicit alterations in DC differentiation. C/EBPβ controls lymphoma-associated DC cytokine expression To assess the contribution of C/EBPβ expression in DCs to lymphoma pathogenesis, we isolated splenic DCs (CD11c + I-A b+ , Fig. 3a , sketch; Supplementary Fig. 3a ) from lymphoma Wt and C/EBP β −/− recipients. DC-derived RNA from tumour-challenged mice was extracted on days 10–13 when enlarged inguinal lymph nodes became palpable and compared with that of naive mice from both genotypes. Applying quantitative real-time PCR (qRT–PCR) arrays, we focused on genes that were informative for immunoregulatory and proliferative processes. Upon tumour challenge, DCs of Wt recipients strongly upregulated gene expression for C/EBP β , IFN -γ , IL-6, IL-10, CCL1, CCL5 and C3 , whereas the transcription factor c-Fos was downregulated. In contrast, DCs from C/EBP β −/− mice failed to upregulate any of the immunomodulatory genes ( Fig. 3a ). In addition, in Wt DCs, a second set of genes was upregulated, including insulin-like growth factor ( IGF-1 ), fibroblast growth factor and hepatocyte growth factor ( HGF ; Fig. 3b ). IGF-1 has been characterized as a growth factor in several tumour entities [20] . Of specific interest is its role in human B-cell precursor acute lymphoblastic leukaemia that shares phenotypic features with the murine E μ -Myc model [21] . Applying a Taqman qRT–PCR assay in DCs derived from tumour-naive C/EBP β −/− mice, we obtained essentially no gene expression for IGF-1 . However, upon lymphoma challenge IGF-1 gene expression was induced ( Fig. 3c ). Correspondingly, E μ -Myc lymphoma cells carried the cell surface receptors for IGF-I, IL-10, IFN-γ and IL-6, whereas the HGF-receptor c-Met was only modestly expressed ( Fig. 3d , Supplementary Fig. 3b ). 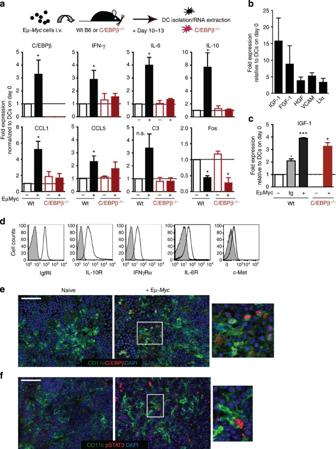Figure 3: C/EBPβ controls inflammatory cytokine release in DCs. (a) RT–qPCR arrays were performed with RNA extracted from splenic DCs isolated from tumour-naive Wt (B6) andCD11c.Cre × C/EBPβflox/flox(C/EBPβ−/−) animals or from Wt andC/EBPβ−/−lymphoma cell recipients 10 and 13 days after tumour challenge (n>10 mice per group;n=3–5 independent experiments). Altered gene expression levels are depicted asx-fold expression normalized to DCs from untreated Wt mice set arbitrarily at 1 (solid horizontal line). Bars represent means±s.e.m.; a Mann–Whitney test was used; *P<0.05. (b) RT–qPCR arrays were performed with RNA extracted from splenic DCs isolated from tumour-naive Wt (B6) and Wt lymphoma cell recipients 10–13 days after tumour challenge (n=10 mice per group;n=2 independent experiments). Altered gene expression levels for genes involved in growth control and adhesion were depicted asx-fold expression normalized to DCs from untreated Wt mice. (c) Single gene-focused RT–qPCR forIGF-1expression in DCs from naive versus lymphoma B-cell-challenged Wt orC/EBPβ−/−mice is presented as for the arrays (DCs from two to three animals were pooled per genotype). Inb,c, bars represent means±s.e.m.; a Student’st-test was applied. *P<0.05; ***P<0.001. (d) Surface expression of cytokine receptors onEμ-Myclymphoma B cells (B220+;n=3–5 independent clones per marker; isotype control, shaded curve). One representative histogram for each cytokine receptor is shown. (e) Spleen sections of naive (n=2) and tumour-challenged mice (days 9–11;n=4) stained for CD11c+DCs, C/EBPβ+and DAPI. A representative section of each group and an enlarged inlet of the boxed area are shown on the right. (f) Spleen sections as inestained for CD11c+, pSTAT3+and DAPI. A representative section of each group is shown. Scale bars, 100 μm. Figure 3: C/EBPβ controls inflammatory cytokine release in DCs. ( a ) RT–qPCR arrays were performed with RNA extracted from splenic DCs isolated from tumour-naive Wt (B6) and CD11c.Cre × C/EBP β flox/flox ( C/EBP β −/− ) animals or from Wt and C/EBP β −/− lymphoma cell recipients 10 and 13 days after tumour challenge ( n >10 mice per group; n =3–5 independent experiments). Altered gene expression levels are depicted as x -fold expression normalized to DCs from untreated Wt mice set arbitrarily at 1 (solid horizontal line). Bars represent means±s.e.m. ; a Mann–Whitney test was used; * P <0.05. ( b ) RT–qPCR arrays were performed with RNA extracted from splenic DCs isolated from tumour-naive Wt (B6) and Wt lymphoma cell recipients 10–13 days after tumour challenge ( n =10 mice per group; n =2 independent experiments). Altered gene expression levels for genes involved in growth control and adhesion were depicted as x -fold expression normalized to DCs from untreated Wt mice. ( c ) Single gene-focused RT–qPCR for IGF-1 expression in DCs from naive versus lymphoma B-cell-challenged Wt or C/EBP β −/− mice is presented as for the arrays (DCs from two to three animals were pooled per genotype). In b , c , bars represent means±s.e.m. ; a Student’s t -test was applied. * P <0.05; *** P <0.001. ( d ) Surface expression of cytokine receptors on Eμ-Myc lymphoma B cells (B220 + ; n =3–5 independent clones per marker; isotype control, shaded curve). One representative histogram for each cytokine receptor is shown. ( e ) Spleen sections of naive ( n =2) and tumour-challenged mice (days 9–11; n =4) stained for CD11c + DCs, C/EBPβ + and DAPI. A representative section of each group and an enlarged inlet of the boxed area are shown on the right. ( f ) Spleen sections as in e stained for CD11c + , pSTAT3 + and DAPI. A representative section of each group is shown. Scale bars, 100 μm. Full size image When we used an enzyme-linked immunosorbent assay (ELISA) for the analysis of supernatants from phorbol myristate acetate (PMA)/ionomycin-stimulated E μ -Myc lymphoma B cells ( n =4 clones tested), no secreted HGF was detectable, which may preclude an autostimulatory loop (data not shown). In support of a tumour-associated upregulation of C/EBPβ in DCs, we frequently detected a specific C/EBPβ nuclear staining in tumour-exposed DCs but not in naive DCs ( Fig. 3e ). In addition, tumour-derived factors can induce the hyperactivation of the JAK2/STAT3 pathway, which results in an abnormal DC differentiation and loss of immunostimulatory capacity in cancer [22] , [23] . STAT3 is normally a latent cytoplasmic transcription factor activated and phosphorylated in response to growth factors and cytokines, such as IL-10 and IL-6. Indeed, secreted IL-6 (range 6–12.21 pg ml −1 ) and IL-10 (range 20–93.57 pg ml −1 ) were detected in cell culture supernatants from isolated lymphoma B cells ( n =4 clones tested), stimulated for 4 h with PMA/ionomycin. As an established marker of tumour-induced changes in DC differentiation and maturation, we observed a substantial number of nuclear-localized phospho-STAT3 + DCs in lymphoma-challenged mice in situ , which was not the case for naive mice ( Fig. 3f ). In vitro treatment of E μ -Myc lymphoma B cells with the STAT3 inhibitor JSI-124 and co-cultured with DCs resulted in essentially complete tumour cell apoptosis ( Supplementary Fig. 3c ), an effect that has also been reported for human ABC-like diffuse large B-cell lymphomas [24] . When E μ -Myc lymphoma-challenged mice were treated for six consecutive days with JSI-124, a delayed clinical disease progression was seen. Although the main growth-inhibitory effect of STAT3 inhibition in all likelihood is directed against tumour cells themselves, we studied maturation phenotypes of DCs from these mice. The most striking reversal of the lymphoma-associated DC maturation defect was obtained in the resident CD11c + CD8 + DC CD205 + subset, since tumour-naive and JSI-124-treated tumour-bearing mice exhibited similar frequencies ( Supplementary Fig. 3d ). Collectively, these observations suggested that the transcriptional activities of STAT3 and C/EBPβ could control DC differentiation and activation upon lymphoma challenge, possibly in a cooperative manner. Lymphoma-educated DCs inhibit T-cell responses in vivo To assess the capacity of E μ -Myc lymphoma-challenged mice to stimulate antigen-specific T-cell proliferation in vivo , we transplanted Wt mice with lymphoma B cells (day 0), followed by the adoptive transfer of eFluor670-labelled CD4 + OT-II T cells on days 7–9. Three days after immunization with the cognate antigen ovalbumin (OVA) in combination with CpGs, the proliferation rate was determined with eFluor670 dilution of transgenic CD4 + T cells ( Fig. 4a,b ). In tumour-bearing mice, reduced frequencies (Wt naive, 1.31±0.24%; Wt+ E μ -Myc , 0.55±0.25%; C/EBP β −/− + E μ -Myc , 1.24±0.20%; mean±s.e.m.) of proliferating T cells were obtained compared with tumour-naive mice. Adoptively transferred OT-II T cells differentiated less efficiently into an IFN-γ + effector phenotype; however, this effect was not statistically significant ( Supplementary Fig. 4a,b ). 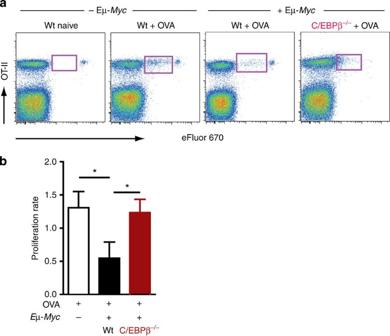Figure 4: Lymphoma DCs mediate the suppression of T-cell responses. (a) Wt mice (B6,n=13) orC/EBPβ−/−mice (n=6) were transplanted with 2 × 105Eμ-Myclymphoma B cells (n=2–3 independent experiments per genotype). Between days 7 and 9, eFluor 670-labelled naive CD4+OT-II T cells (6–8 × 105) were adoptively transferred into tumour-bearing mice or tumour-naive mice (n=9). Mice were immunized by s.c. injection of 100 μg OVA protein and 25 μg CpGs. Control Wt andC/EBPβ−/−animals received T cells but no OVA protein. Proliferation of transferred T cells in draining lymph nodes was analysed with flow cytometry on day 3. Representative FACS plots of gated CD4+cells from draining lymph nodes are shown; numbers indicate the percentage of proliferated OVA-specific CD4+/OT-II+/eFluor670+T cells in recipient mice within the gate. (b) Quantification of the proliferation rate. Bars represent means±s.e.m.; a Student’st-test was used. *P<0.05. Figure 4: Lymphoma DCs mediate the suppression of T-cell responses. ( a ) Wt mice (B6, n =13) or C/EBP β −/− mice ( n =6) were transplanted with 2 × 10 5 Eμ-Myc lymphoma B cells ( n =2–3 independent experiments per genotype). Between days 7 and 9, eFluor 670-labelled naive CD4 + OT-II T cells (6–8 × 10 5 ) were adoptively transferred into tumour-bearing mice or tumour-naive mice ( n =9). Mice were immunized by s.c. injection of 100 μg OVA protein and 25 μg CpGs. Control Wt and C/EBP β −/− animals received T cells but no OVA protein. Proliferation of transferred T cells in draining lymph nodes was analysed with flow cytometry on day 3. Representative FACS plots of gated CD4 + cells from draining lymph nodes are shown; numbers indicate the percentage of proliferated OVA-specific CD4 + /OT-II + /eFluor670 + T cells in recipient mice within the gate. ( b ) Quantification of the proliferation rate. Bars represent means±s.e.m. ; a Student’s t -test was used. * P <0.05. Full size image Next, considering the influence of the transcription factor C/EBPβ on the immunosuppressive properties of MDSCs, we first compared the priming capacity of bone marrow (BM)-derived DCs from Wt and C/EBP β −/− mice using a co-culture system. In this assay, DCs were pulsed with an OVA-peptide (aa 323–339), and proliferation of OT-II T cells was measured 3 days later with eFluor670 dilution. The stimulatory capacity of C/EBP β-deleted DCs in this in vitro system was unimpaired ( Supplementary Fig. 4c,d ). To address the role of C/EBP β in vivo , mice with the DC-specific deletion were E μ -Myc lymphoma-transplanted and further treated as for Wt recipients ( Fig. 4a,b ). In these mice, OT-II T cell proliferation was reverted and comparable to naive mice ( Fig. 4b ), suggesting that C/EBPβ is involved in a DC-inherent immunosuppressive programme. C/EBPβ expressing DCs stimulate lymphoma B-cell survival To dissect the mechanisms of DCs in supporting lymphoma pathogenesis, we co-cultured E μ -Myc lymphoma cells and BM-derived myeloid DCs. In vitro , DCs strongly supported the viability (Annexin V − 7-AAD − ) of lymphoma cells ( Supplementary Fig. 5a,b ). Additional inclusion of the CCR7 ligands CCL19 and CCL21, which FRCs express, had only moderate effects compared with DCs alone. To address the question whether DC-provided pro-survival signals rely on the activity of C/EBPβ, we co-cultured Wt myeloid DCs, C/EBP β −/− DCs and E μ -Myc lymphoma cells, respectively. In contrast to Wt DCs, C/EBP β −/− DCs exhibited a significantly lower capacity to rescue E μ -Myc lymphoma cells from apoptosis (Annexin V + 7-AAD + ) ( Fig. 5a , Supplementary Fig. 5b ). 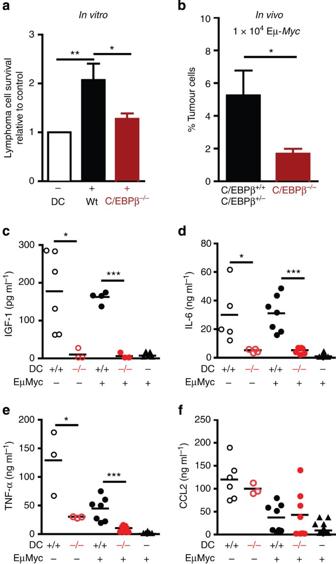Figure 5: DCs expressing C/EBPβ antagonize apoptosis in lymphoma cells. (a)Eμ-Myctumour cells were co-cultured with Wt BM myeloid DCs orC/EBPβ−/−DCs (B6). Lymphoma cell survival was determined as inSupplementary Fig. 5a,b(n=5 individual Eμ-Myccell clones tested). Data are presented as fold change in lymphoma cell survival in the presence of DCs versus absence of DCs. Bars represent means±s.e.m.; a Student’st-test was used. *P<0.05; **P<0.01. (b)C/EBPβ−/−mice and Wt or heterozygous littermates as controls were challenged with 1 × 104Eμ-MycGFP cells i.v. Tumour load in spleens ofC/EBPβ−/−(n=5) compared with controls (n=6) was assessed with flow cytometry on day 7 (n=2 independent experiments). (c–f) Culture supernatants were obtained from co-cultures as ina, followed by determination of cytokine content in cytokine bead arrays. Inb–f, bars represent means±s.e.m.; a Mann–Whitney test was applied. *P<0.05; **P<0.01; ***P<0.001. Figure 5: DCs expressing C/EBPβ antagonize apoptosis in lymphoma cells. ( a ) Eμ-Myc tumour cells were co-cultured with Wt BM myeloid DCs or C/EBP β −/− DCs (B6). Lymphoma cell survival was determined as in Supplementary Fig. 5a,b ( n =5 individual Eμ- Myc cell clones tested). Data are presented as fold change in lymphoma cell survival in the presence of DCs versus absence of DCs. Bars represent means±s.e.m. ; a Student’s t -test was used. * P <0.05; ** P <0.01. ( b ) C/EBP β −/− mice and Wt or heterozygous littermates as controls were challenged with 1 × 10 4 Eμ-Myc GFP cells i.v. Tumour load in spleens of C/EBP β −/− ( n =5) compared with controls ( n =6) was assessed with flow cytometry on day 7 ( n =2 independent experiments). ( c – f ) Culture supernatants were obtained from co-cultures as in a , followed by determination of cytokine content in cytokine bead arrays. In b – f , bars represent means±s.e.m. ; a Mann–Whitney test was applied. * P <0.05; ** P <0.01; *** P <0.001. Full size image Next, to assess the influence of C/EBP β-deficient DCs on lymphoma growth in vivo , we challenged C/EBP β −/− , C/EBP β +/+ or C/EBP β +/− mice with E μ -Myc lymphoma B cells. CD11c + cell-selective deletion of C/EBP β significantly retarded lymphoma progression in the spleen ( Fig. 5b ). Growth-promoting factors that are not known to be C/EBPβ-dependent could be released by DCs and contribute to E μ -Myc lymphoma progression [25] . Here we detected protein expression of indian hedgehog (Ihh) in isolated DCs from naive and tumour-bearing mice ( Supplementary Fig. 5c ). Likewise, BM-derived C/EBP β −/− DCs showed abundant expression of this growth factor ( Supplementary Fig. 5c ). Pertussis toxin (Ptx) acts on the Smoothened (Smo) receptor in the hedgehog survival pathway; inclusion of this drug considerably diminished lymphoma B-cell survival in DC co-cultures ( Supplementary Fig. 5d ). This finding was consistent with the specific inhibitory effect of the Smo-inhibitor cyclopamine in this co-culture system ( Supplementary Fig. 5e ) [26] . Thus, DCs contribute by a paracrine signalling mechanism to a stromal network that nurtures lymphoma B cells. In vitro , E μ -Myc lymphoma B cells undergo rapid apoptosis in the absence of stromal support, a property shared with human acute lymphoblastic leukaemia cells and other lymphomas [27] . To assess the pro-survival effect of single cytokines or their combination, freshly isolated E μ -Myc lymphomas were co-cultured with irradiated NIH3T3 cells and further supplemented with cytokines expressed in the T-cell zone of SLOs ( Supplementary Fig. 6a ). We examined five different clones for their survival (Annexin V − 7-AAD − ) in the presence of the indicated cytokines. Although each of these cases showed gain of viability upon a mixture or some specific cytokines, it appeared that these clones had differential requirements for survival. Release of pro-inflammatory and immunoregulatory cytokines from DCs could also contribute to the formation of a growth-promoting milieu in lymphoma and results in a T-cell antigen unresponsiveness. Here we assessed secretion of the key cytokines and chemokines in supernatants from Wt myeloid DCs, C/EBP β −/− DCs and E μ -Myc lymphoma cell co-cultures. The secretory behaviour of Wt DCs and C/EBPβ-deleted DCs was clearly distinguishable because release of IGF-1, IL-6 and TNF-α from Wt DCs was substantially higher ( Fig. 5c–e ). No differences were observed for IFN-γ, IL-10 or the pro-inflammatory chemokine CCL2 ( Fig. 5f ). In this short-term in vitro co-culture system, inclusion of E μ -Myc lymphoma B cells had no additional effects on the C/EBPβ-controlled secretion of IGF-1 and IL-6 from steady-state resting DCs. The discrepancies between the gene expression profiles ( Fig. 3 ) and the detection of secreted protein ( Fig. 5c–e ) can be best explained by the origin of the DCs. While we obtained gene expression profiles of naive versus tumour-challenged DCs in animals exposed to transplanted tumours for at least 10–13 days, in vitro co-cultures of BM-derived DCs lasted for only 24 h. Next, we also considered pro-inflammatory or immunoregulatory cytokine secretion in transplanted lymphomas because the cytokine-controlled remodelling of the tumour–stroma interface and the T-cell tumour responsiveness could change shortly after lymphoma challenge in vivo . DCs from tumour-naive and lymphoma-transplanted mice were isolated and stimulated with PMA/ionomycin ( Supplementary Fig. 6b ). Corresponding to the RNA data from the adoptive transfer model ( Fig. 3a ), tumour-exposed DCs released IFN-γ, IL-6, IL-10 and IGF-1 in about two- to three–fold higher amounts compared with naive DCs. No differences were observed for CCL2 and TNF-α. Together, cytokine protein expression from DCs in vivo reflects an immunomodulatory condition and indicates that our tumour transfer model recapitulates a DC-associated alteration of the immune microenvironment. In this process, C/EBPβ plays a leading role. Differentiation of DCs in the absence of C/EBPβ C/EBPβ is known to control emergency granulopoiesis induced by cytokines and infections [28] . To rule out that lineage-specific deletion of C/EBP β during myelopoiesis could result in aberrant DC differentiation, we analysed in vitro cultured BM-derived DCs from Wt and C/EBP β −/− mice. Within 7 days, precursor cells from both genotypes matured similarly under either GM-CSF only or GM-CSF+IL-4+TNF-α stimulation conditions ( Fig. 6a ). Surface expression of MHC class II and costimulatory molecules and the frequencies of DC (CD11c + CD11b + ), macrophage (CD11c − CD11b + ) and granulocyte (CD11c − Gr-1 + ) myeloid subsets were comparable ( Fig. 6b ), suggesting that C/EBPβ is not essential for the differentiation of myeloid DCs from BM precursors. 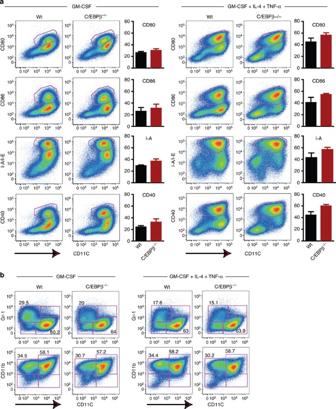Figure 6: DC differentiation can occur in the absence of C/EBPβ. (a) BM cells were cultured for 7 days in the presence of GM-CSF alone, or supplemented with GM-CSF, IL-4 (days 1–7) and TNF-α (days 5–7). Cells differentiated under these distinct culture conditions were analysed on day 7 by flow cytometry for the expression of CD11c and the maturation markers MHC class II (I-A), CD80, CD86 and CD40. Shown are representative dot blots of DCs (CD11c+) and secondary marker expression, gates depict double-positive subsets. Expression levels for these secondary markers are given as the mean fluorescence intensities (MFIs), and graphs depict means±s.e.m. of two independent experiments withn=5 Wt andn=5C/EBPβ−/−animals. (b) BM precursors were cultured for 7 days as ina. Distribution of myeloid subpopulations was analysed with flow cytometry. Gates within the histograms define differentiated myeloid DCs (CD11c+CD11b+). Subsets of CD11c−CD11b+and CD11c−Gr-1+cells represent macrophage and granulocyte differentiation lineages, respectively; numbers indicate the frequencies of subsets within the gates. Representative dot plots are from two experiments withn=4 Wt andn=4C/EBPβ−/−animals. Figure 6: DC differentiation can occur in the absence of C/EBPβ. ( a ) BM cells were cultured for 7 days in the presence of GM-CSF alone, or supplemented with GM-CSF, IL-4 (days 1–7) and TNF-α (days 5–7). Cells differentiated under these distinct culture conditions were analysed on day 7 by flow cytometry for the expression of CD11c and the maturation markers MHC class II (I-A), CD80, CD86 and CD40. Shown are representative dot blots of DCs (CD11c + ) and secondary marker expression, gates depict double-positive subsets. Expression levels for these secondary markers are given as the mean fluorescence intensities (MFIs), and graphs depict means±s.e.m. of two independent experiments with n =5 Wt and n =5 C/EBP β −/− animals. ( b ) BM precursors were cultured for 7 days as in a . Distribution of myeloid subpopulations was analysed with flow cytometry. Gates within the histograms define differentiated myeloid DCs (CD11c + CD11b + ). Subsets of CD11c − CD11b + and CD11c − Gr-1 + cells represent macrophage and granulocyte differentiation lineages, respectively; numbers indicate the frequencies of subsets within the gates. Representative dot plots are from two experiments with n =4 Wt and n =4 C/EBP β −/− animals. Full size image LAP/LAP* expression is associated with lymphoma growth Three isoforms of C/EBPβ with different N-terminal lengths have been described. In general, the liver-enriched activator protein (LAP)/LAP* isoforms are associated with a transcriptionally active state, whereas the short isoform liver-enriched inhibitor protein (LIP) lacking the transactivation domain rather acts as a repressor. However, LIP can also serve as a transcriptional activator depending on the cellular context. The C/EBPβ isoform ratio is mainly controlled by mTOR signalling, which affects the activity of the translation initiation factor eIF4E, which in turn is involved in C/EBPβ isoform switching [29] , [30] . To analyse whether Eμ- Myc lymphoma B cells influence C/EBPβ isoform ratios in DCs, we retrieved splenic DCs (CD11c + I-A b+ , Supplementary Fig. 3 ) from naive and tumour-challenged Wt mice. In immunoblot analysis, the LAP/LAP*:LIP ratio in tumour-exposed DCs increased about 2.5-fold compared with tumour-naive DCs ( Fig. 7a,b ; Supplementary Fig. 8 ). We conclude that E μ -Myc lymphoma residency in SLOs launches a process that is characterized by the upregulation of the transcription factor C/EBPβ in DCs. Moreover, the challenge with lymphoma B cells in vivo favours the alternative translation of C/EBPβ isoforms in DCs. 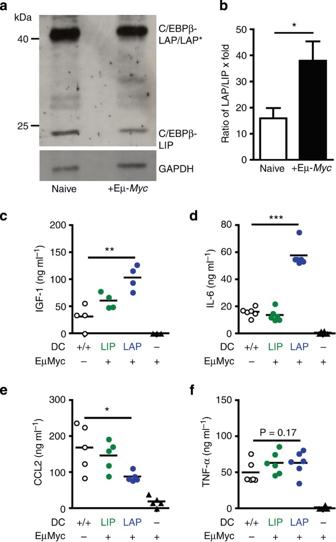Figure 7: Lymphoma-derived factors control C/EBPβ isoform ratios. DCs from naive and tumour-challenged mice (days 7–10) were isolated as inFig. 3a, and protein lysates were analysed using SDS–PAGE and immunoblotting. (a) All three isoforms of C/EBPβ were detected with anti-C/EBPβ antibody, and anti-GAPDH was used as loading control. Images have been cropped for presentation; a full size image is presented inSupplementary Fig. 8. (b) The ratios of LAP/LAP* to LIP were determined by densitometric scanning and are expressed as bar graphs (n=4 independent experiments, with >n=20 mice per group). Bars represent means±s.e.m., a Mann–Whitney test was applied. (c–f) Myeloid DCs from Wt,LIPandLAPknock-in mice were generated and co-cultured as inFig. 5awithEμ-Myclymphoma B cells, and culture supernatants were analysed by cytokine bead array or ELISA inFig. 5c–f. Graphs depict means. *P<0.05; **P<0.01; ***P<0.001. A Mann–Whitney test was applied. Figure 7: Lymphoma-derived factors control C/EBPβ isoform ratios. DCs from naive and tumour-challenged mice (days 7–10) were isolated as in Fig. 3a , and protein lysates were analysed using SDS–PAGE and immunoblotting. ( a ) All three isoforms of C/EBPβ were detected with anti-C/EBPβ antibody, and anti-GAPDH was used as loading control. Images have been cropped for presentation; a full size image is presented in Supplementary Fig. 8 . ( b ) The ratios of LAP/LAP* to LIP were determined by densitometric scanning and are expressed as bar graphs ( n =4 independent experiments, with > n =20 mice per group). Bars represent means±s.e.m., a Mann–Whitney test was applied. ( c – f ) Myeloid DCs from Wt, LIP and LAP knock-in mice were generated and co-cultured as in Fig. 5a with Eμ-Myc lymphoma B cells, and culture supernatants were analysed by cytokine bead array or ELISA in Fig. 5c–f . Graphs depict means. * P <0.05; ** P <0.01; *** P <0.001. A Mann–Whitney test was applied. Full size image As C/EBPβ isoforms might display contrasting functions in gene activation depending on the contextual framework, we generated BM-derived DCs from LAP/LAP* ( Δ uORF) and LIP knock-in mice [31] , [32] . LAP/LAP* knock-in DCs released a considerably higher amount of IGF-1 and IL-6 as compared with Wt or LIP isoform DCs ( Fig. 7c,d ). Conversely, CCL2 release from LAP/LAP* knock-in DCs was diminished compared with LIP knock-in and Wt DCs ( Fig. 7e ). Substantial evidence indicates pathogenic functions for IL-6 in various tumours [33] . Depending on the model system, the JAK2/STAT3 pathway is either a downstream target or, conversely, might be involved in the upstream regulation of IL-6 expression and secretion [34] . As crosstalk between the two IL-6 transcriptional regulators NF-κB and C/EBPβ has been described, we measured NF-κB protein–DNA-binding activity in Wt and CEBP β −/− DCs by the electrophoretic mobility shift assay. We found that in unstimulated ( Supplementary Fig. 7a ) and in lipopolysaccharide-stimulated ( Supplementary Fig. 7b ) DCs, NF-κB DNA-binding activity was largely unchanged, regardless of the C/EBPβ status of the cells, suggesting that alterations in cytokine expression cannot be attributed to modifications in NF-κB activity. In this report, we show that DCs can condition the environment of SLOs and provide pro-survival signals to a rapidly progressing Myc-driven B-cell lymphoma. The transcription factor C/EBPβ governs this capacity of DCs, which acts in concert with a C/EBPβ-associated creation of a tumour-induced immunosuppression programme. We demonstrate that in vivo depletion of DCs resulted in an impaired E μ -Myc lymphoma growth in mice, a finding that is consistent with the occurrence of a lymphoma-imposed modulation of DC maturation. There is ample evidence that the function of DC subsets in spontaneous or transplanted tumours is dependent on maturation and activation status of DCs [4] , [35] , [36] . In E μ -Myc transgenic mice that exhibit a large tumour mass, a decrease in the activating costimulatory molecule CD40, loss of MHC class II, and an increase in CD80 and PD-L1 was observed. Expression of PD-L1 as a negative regulator of T-cell activation could contribute to deficient T-cell stimulatory capacity and, thus, support tumour-induced tolerance [37] . In the transplantable lymphoma model, which we have chosen to recapitulate early phases of lymphoma expansion, we obtained an alteration of CD11c + subset composition including loss of mature DCs (CD4 + /CD11c high ), and a reduction in the resident CD11c + /CD8 + /CD205 + DC subpopulation. CD205 functions as a receptor for CpG oligodeoxynucleotides, and its deficiency leads to impaired DC maturation, an inability to make IL-12, and a reduction in T-cell stimulatory capacity [17] , [18] . Collectively, lymphoma-resident DCs could be compromised in their capacity to capture and present antigens to T cells. However, the consideration of costimulatory markers alone seems insufficient to predict the capacity of DCs for T-cell priming in vivo . In many solid tumour models it has been shown that suppression of DC function and subset composition is often mediated by tumour cells themselves, MDSCs, macrophages or tumour-infiltrating lymphocytes [3] , which produce an abundance of deleterious cytokines, chemokines and growth factors. Several tumour-derived factors could have an impact on the myeloid cell composition of the tumour microenvironment. More specifically, vascular endothelial growth factor, M-CSF, GM-CSF, IL-10, IL-6, PGE2, transforming growth factor-β1 and gangliosides were suggested to impair DC differentiation and functionality [38] . Although an extensive screen for lymphoma-derived factors is beyond the scope of this work, we confirmed secretion of IL-6 and IL-10 by Eμ- Myc lymphoma B cells. Both factors are of particular interest because they can induce either STAT3 phosphorylation or C/EBPβ expression from DCs [16] , [38] . Here we used the detection of pSTAT3 primarily as a biomarker for lymphoma-associated activation in DCs. Recently, a link was reported between STAT3 and CEPB/β [39] in regulating myelopoiesis. In tumours both factors support the differentiation of MDSCs [38] . In DCs it has been shown that C/EBPβ and STAT3 share several activation pathways, foremost the expression of pro-inflammatory cytokines and maturation markers. In hepatocytes, STAT3 activation is essential for IL-6-mediated C/EBP β gene transcription through activation and tethering of STAT3 to the promoter region [40] . In our work we focused on the conditions that are shaped by lymphoma-challenged DCs and that could influence either direct tumour growth or the formation of a tolerogenic environment. Enhanced expression of cytokines and chemokines involved in the formation of a pro-inflammatory milieu, including IL-6, CCL1 and CCL5, could relate to the development of a tumour-permissive niche, as has been suggested for human Hodgkin lymphoma [41] . Furthermore, increased availability of IL-10 might contribute to the conditions for developing an immunosuppressive state [42] , [43] . IL-10 can either act on APCs through inhibiting costimulatory molecule and MHC expression, or downregulates the secretion of T helper1 cytokines and induces T regulatory responses. Regarding human lymphoma biology, IL-10 expression is thought to promote the development of Burkitt’s lymphoma through production of the B-cell growth-promoting cytokine BAFF. In accordance, in patients suffering from diffuse large B-cell lymphoma, elevated BAFF serum levels were detected and correlated with poor prognosis [44] . IGF-1 has been suggested to serve as B-cell leukaemia growth factor [21] , [45] ; here it was released from tumour-naive and tumour-exposed Wt DCs, in vitro and in vivo . As expected, IGF-1 gene expression from tumour-naive C/EBP β −/− DCs was very low [46] , whereas lymphoma-conditioned DCs upregulated the IGF-1 gene message substantially. We conclude that transcriptional activators other than C/EBPβ could contribute to IGF-1 transcriptional regulation, depending on tumour-imposed stress conditions. Indeed, several other transcription factors were shown to activate IGF-1 transcription in diverse cell types, including Stat5 in hepatocytes and putatively in DCs [47] , [48] , [49] , C/EBPδ in osteoblasts and putatively DCs [50] , and IRF8 in hepatocytes [51] . When IGF-1 and other potentially B-cell growth-promoting cytokines were tested in a DC-independent cell culture, gain of viability between the E μ -Myc lymphoma B-cell clones varied substantially. Such variation is frequently observed among primary leukaemia or lymphoma cases in human, probably reflecting individual genetic mutations that result in apoptosis resistance or proliferation signalling [27] , [52] . Gene expression of HGF in tumour-conditioned DCs would be consistent with the role of the c-Met ligand in the integrin-mediated adhesion of B cells to both VCAM-1 and fibronectin, which could also favour migration and adhesion of E μ -Myc lymphoma B cells within SLOs [53] , [54] . Alternatively, since c-Met expression in E μ -Myc lymphoma B cells was low, we envision that HGF could gain instead a tumour-promoting role through the auto- or paracrine inhibition of DC function and promotion of IL-10-producing regulatory T-cell differentiation, as shown in central nervous system autoimmune models [55] . DC-mediated pro-survival effects were strongly dependent on a Ptx-sensitive, Gαi-coupled signalling pathway. This finding relates to the efficiency of the Smo-inhibitor cyclopamine and reveals the relevance of the hedgehog pathway for the survival of E μ -Myc lymphoma B cells [14] , [25] . Here we demonstrate that DCs can provide Ihh to lymphoma B cells. In this pro-survival signalling process, Ihh binds to its receptor Patched 1, which leads to its inactivation. Subsequently, Patched 1 can no longer inhibit the Gαi-coupled receptor Smo. Smo activation normally triggers the activation of GLI transcription factors, which regulate target genes in tumour cell growth and survival [56] . Inhibition of hedgehog signalling has emerged as a druggable target in clinical tumour trials [57] . We suggest that the alteration of DC differentiation in conjunction with a strong induction of pro-inflammatory cytokines and growth factors supports the hypothesis that lymphoma B cells co-opt stromal DCs to their own growth advantage. How is this crosstalk between lymphoma B cells and DCs regulated? While the influence of NF-κB, STAT and AP-1 signalling in context of a pro-tumoral inflammatory reaction in solid tumour models has been appreciated [58] , [59] , the role of C/EBPβ in these processes remained incompletely understood. For MDSCs and tumour-associated macrophages in solid tumours, a contextual regulation of C/EBPβ activity favouring an immunosuppressive environment has been suggested [16] , [60] . In the aggressive E μ -Myc lymphoma model, the transcription factor C/EBPβ has the principal role in shaping a DC-dependent formation of a pro-inflammatory and growth-promoting milieu in SLOs. Lymphomagenesis differs substantially from the immunosuppressive programme characteristic of several solid tumours because expansion of Eμ -Myc lymphomas proceeds very rapidly in a lymph node environment that is optimized for B lymphocyte ontogeny [61] . To study the consequences of an altered DC-mediated immune regulation in Eμ- Myc lymphoma, tumour-bearing animals were adoptively transferred with OT-II T cells. In Wt animals, a reduction in T-cell proliferation and in IFN-γ-producing effector T cells suggested that lymphoma growth imposes an immunosuppressive programme. The lineage-specific ablation of C/EBP β reverted this tumour-induced tolerance. Hence, C/EBPβ inhibition could serve as a target gene function for reinstalling T-cell responsiveness. In human it has been shown that T-cell-mediated immune responses against c-Myc-positive B-cell lymphomas are only weakly elicited [62] . It remains to be shown whether DC-mediated modulation of the adaptive T-cell response towards a Myc-driven tumour can exert a dominating tumour-promoting or -inhibiting effect. The lymphoma-associated programme in DCs is highlighted by the induction of C/EBPβ and the preferential translation of the LAP/LAP* C/EBPβ isoform. This isoform shift could also reflect DC differentiation processes leading to a specific gene transcription pattern [32] . While a complete identification of lymphoma-derived factors that act on DC differentiation requires further investigation, we show that shifting the C/EBPβ isoform ratio in favour of LAP/LAP* is consistent with the preferential expression of the pro-inflammatory cytokine IL-6 (ref. 63 ) and the growth factor IGF-1 in DCs [21] , [45] , [46] . Unexpectedly, CCL2 secretion from LIP knock-in DCs was similar to Wt DCs [64] , indicating that LIP might have a role in transcriptional activity beyond its function as a repressor. An alternative explanation for the diminished secretion of CCL2 from LAP knock-in DCs includes a repressor activity of this isoform; however, it remains to be shown how the absence of the competing LIP region affects the transcriptional activity on the CCL2 promoter in a cell-type-specific manner [65] . We propose that the encounter between E μ -Myc lymphoma B cells and DCs can mimic an early pathogenic condition. Upon arrival of transformed B cells in SLOs, Myc-driven lymphoma cells lodge within a microenvironment that counteracts their inherent apoptosis programme. In this scenario, DCs play a leading role, provided that they express C/EBPβ. We extend the role of this transcription factor to the generation of a tumour-permissive niche, and thus establish a previously unidentified reciprocal relationship between DC functions and lymphomagenesis. From our findings, a clinical implication emerges. Immunomodulatory derivatives of thalidomide mediate part of their antiproliferative effect through downregulation of C/EBPβ expression in multiple myeloma cells [8] . Although a concurrent impact of these drugs on stromal cells remained unexplored, we envision that targeting C/EBPβ in DCs could complement traditional cytotoxic therapies for the cure of Myc-driven B-cell lymphoma. Mice E μ -Myc (C57BL/6) transgenic mouse breeder pairs [66] were obtained from Jackson Laboratories (Bar Harbor, ME, USA), C57BL/6 (CD45.1 + ) congenic breeder pairs were from Taconic Farms (Denmark) and C57BL/6 mice were obtained from Charles River (Sulzfeld, Germany), if not stated otherwise. The CD11c.DOG transgenic mouse strain on a C57BL/6 background was obtained from N. Garbi [67] . The C/EBP β flox/flox transgenic mouse strain was backcrossed into the CD11c.Cre transgenic mouse strain (C57BL/6 strain background) (Jackson Laboratories) to generate CD11c.Cre x C/EBP β flox/flox mice; this strain is referred to as C/EBP β −/− throughout the manuscript. The LIP and C/EBP β Δ uORF knock-in mice have been described earlier [31] , [32] ; this latter strain is also referred to as LAP*/LAP knock-in mouse throughout the manuscript. The genetic background of these mice was C57BL/6 × 129Ola. Control groups of Wt mice were always matched for age and strain background. In all adoptive tumour cell transfers, recipient mice were used at the age of 7–12 weeks, and groups were sex-matched according to the origin of the donor E μ -Myc clone. Tumour clones from male and female donors were used. All animal studies were performed according to the institutional and Berlin State guidelines (approved by the Landesamt für Gesundheit und Soziales, Berlin; registered under LaGeSo 0371/05 and 0333/06). Cell culture and apoptosis of primary E μ -Myc lymphoma cells E μ -Myc transgenic mice were monitored for signs of disease, which includes development of palpable lymphomas or weight loss of more than 20%. Lymph node-derived lymphoma cell suspensions were prepared from diseased mice by tissue homogenization. For DC-lymphoma cell co-cultures, BM-derived DCs from C57BL/6 mice were generated. BM cells were obtained by flushing femur and tibia with RPMI medium. Cells were cultured at 2 × 10 5 ml −1 in RPMI 1640 containing 10% (v/v) fetal calf serum (FCS), glutamine, Na-pyruvate, penicillin/streptomycin, β-mercaptoethanol (50 μM) and 20 ng ml −1 GM-CSF (Peprotech). Cells were not further replated and, instead, half of the medium was replaced every second day. On days 7–8 of culture, residual B cells were depleted with Mouse Pan B Dynabeads (Life Technologies), yielding a DC population of >90% CD11c + cells. DCs were seeded into six-well tissue culture plates (1.5 × 10 6 per well), followed by addition of freshly prepared lymphoma cells from diseased mice (5 × 10 6 per well) in lymphoma medium containing RPMI 1640 and IMDM (1:1; PAA Laboratories and Invitrogen) with 10% (v/v) FCS, penicillin–streptomycin, glutamine and Na-pyruvate, supplemented with 25 μM β-mercaptoethanol. CCL19, CCL21 (R&D) were added to the co-cultures at 500 ng ml −1 . Cyclopamine (Sigma) dissolved in dimethylsulphoxide and Ptx (Calbiochem; 0.5 μg ml −1 PBS) were added as specified in Figure legends. After 20–24 h, lymphoma B cells were stained with anti-B220 antibody, and survival was assessed with flow cytometry applying AnnexinV-FITC and 7-AAD staining (eBioscience). Survival was assessed as B220 + /AnnexinV − /7-AAD − , and values were normalized to the survival fraction of lymphoma cells in the absence of DCs (set arbitrarily=1). In each individual experiment, an independent primary E μ -Myc lymphoma cell clone was used. Differentiation of DCs from Wt, CD11c-Cre x C/EBP β flox/flox mice was performed in the presence of GM-CSF only (20 ng ml −1 ), or in medium supplemented with IL-4 (50 U ml −1 ) and TNF-α (50 ng ml −1 ; all from Peprotech). Cells on day 7 were analysed with flow cytometry for maturation markers and cellular subset composition. Generation of a retroviral vector and transduction of lymphoma cells To generate E μ -Myc eGFP transgenic lymphoma cells, the retroviral plasmid pMSCV-IRES-eGFP was transfected into the packaging cell line Plat-E. Retroviral supernatant was harvested and filtered, followed by three rounds of transduction by spinoculation of primary E μ -Myc lymphoma cells, in the presence of 4 μg ml −1 polybrene. Enhanced green fluorescence protein (EGFP)-stained lymphoma cells were further enriched using fluorescence-activated cell sorting (FACS) sorting before transfer into animals. Lymphoma cell transfer C57.BL/6 (CD45.2), C57BL/6 (CD45.1) congenic, CD11c.DOG and CD11c-Cre x C/EBP β flox/flox mice 7–12 weeks of age were injected i.v. with 1 × 10 4 to 2 × 10 5 E μ -Myc lymphoma cells (CD45.2), as indicated. Mice were examined three times per week for lymphoma growth. Onset of disease was defined as palpable tumour nodules, weight loss and paralysis. For transfer of E μ -Myc lymphoma cells into DC-depleted recipient mice, the DT receptor system was used. In CD11c.DOG mice, the DT receptor is under the control of a cloned CD11c promoter [67] . DT (Sigma) injections (3–4 × per week) starting on day −1 (8 ng per g body weight) induced the deletion of DCs (CD11c + ). The efficiency of deletion was confirmed in the spleen and lymph node (LN) using flow cytometry. Preparation of cell suspensions for flow cytometry Spleen and lymph node cell suspensions were obtained by gentle disruption of the organ in PBS/2% (v/v) FCS followed by hypotonic lysis to deplete red blood cells. Cells were blocked with CD16/32 antibody (1:100 diluted) in FACS buffer (PBS, 0,5% (w/v) bovine serum albumin, 0,05% (v/v) NaN 3 ), followed by staining with the specific antibodies as detailed in Figure legends: fluorescein isothiocyanate (FITC), allophycocyanin (APC) and Pacific Blue-labelled rat anti-mouse CD4; FITC, APC and Pacific Blue-labelled rat anti-mouse CD8α; APC-labelled rat anti-mouse B220 (CD45R); Pacific Blue-labelled mouse anti-mouse CD45.2; FITC and Alexa Fluor (AF) 647-labelled mouse anti-mouse I-A b (MHC class II); APC-labelled rat anti-mouse I-A/I-E (1:1,000 dilution); rat anti-mouse CD16/CD32; Phycoerythrin (PE)-labelled rat anti-mouse CD210 (IL-10R); FITC and APC-labelled hamster anti-mouse CD80; FITC and APC-labelled rat anti-mouse CD86; FITC and Alexa Fluor 647-labelled rat anti-mouse CD11b; FITC, Pacific Blue and Alexa Fluor 647-labelled hamster anti-CD11c; Alexa Fluor 647-labelled rat anti-mouse CD205 (1:10; DEC-205); FITC-labelled rat anti-mouse CD40; APC-labelled rat anti-mouse PD-L1 (CD274); biotinylated hamster anti-mouse IFN-γR α chain (CD119); PE- and APC-labelled IL-6R α (1:20; CD126); FITC and Alexa Fluor 647-labelled rat anti-mouse Gr-1 (1:300; Ly-6G/Ly-6C; all from Biolegend); chicken anti-mouse Igf-IR (Abcam); biotinylated hamster anti-mouse gp38 (eBioscience); FITC-coupled rat anti-mouse Vα2 TCR (OT-II); PE-labelled goat anti-rat IgG (1:200); APC-, PerCP- or PE-labelled streptavidin (all from BD Biosciences); rabbit anti-mouse c-Met (1:20; sc-161, Santa Cruz); and Cy5-labelled donkey anti-chicken IgY (Jackson ImmunoResearch). All antibodies were used in a 1:100 dilution in FACS buffer, except for those specified in the list. Data were acquired on a FACSCantoII flow cytometer (Becton Dickinson) and were further analysed with the FlowJo software (TreeStar). Cell sorting was carried out on a FACSAria (Becton Dickinson). Immunohistology For frozen sections, tissues were frozen in Tissue Tek OCT compound (Sakura Finetek). Cryosections of 6-μm thickness were cut, air-dried and fixed for 10 min in −20 °C acetone. For immunofluorescence, sections were blocked for 30 min with 10% (v/v) normal mouse or goat serum, respectively; slides were stained for 1.5 h at room temperature with biotinylated or fluorescently labelled antibodies: Alexa Fluor 488- and Alexa Fluor 647-labelled hamster anti-mouse CD11c; Pacific Blue-labelled mouse anti-mouse CD45.2 (Biolegend); hamster anti-mouse gp38 (eBioscience); biotinylated hamster anti-mouse CD11c (BD Biosciences); rabbit anti-mouse-phosphorylated STAT3 (1:100 dilution; Tyr705; Cell Signaling); rabbit anti-mouse CCL21 (R&D); biotinylated rat anti-mouse CD21/CD35 antibody (1:250; Biolegend). Secondary antibody included the following: goat anti-rabbit Alexa Fluor 568 (1:200) and goat anti-hamster Alexa Fluor 568 (Molecular Probes). All antibodies were used in a 1:50 dilution in PBS, except for those specified in the list. Biotinylated primary antibodies were detected with streptavidin Alexa Fluor (AF) 488 or −568 (Molecular Probes; 1:200–1:400). All slides were mounted in Mowiol solution. For the detection of phosphorylated STAT3 (pSTAT3, Tyr 705), sections were sequentially fixed in acetone for 10 min, and then in methanol for further 10 min at −20 °C. All incubation and washing steps were performed in Tris-NaCl buffer (pH 7.6). Sections were blocked for 30 min with normal goat serum, and then stained for 3 h with rabbit anti-mouse pSTAT3 at room temperature. For the detection of unconjugated rabbit antibody, secondary goat anti-rabbit AF568 antibody was incubated for another 1 h. DCs were stained with hamster anti-mouse CD11c AF488 for 1 h, and finally nuclei were detected with 4′,6-diamidino-2-phenylindole (DAPI). C/EBPβ was detected with an antibody (clone 1H7, Biolegend) that recognizes all three isoforms. DCs and nuclei were co-stained as described. Briefly, acetone-fixed slides from lymph nodes derived from naive B6 mice, lymphoma-bearing mice on days 6, 7 or 9 were fixed in acetone. Sections were blocked for 30 min in normal mouse serum (10% v/v), followed by an incubation with mouse anti-C/EBPβ biotin (1:100) for 1.5 h, and detection with steptavidin-AF568 (1:200) for another 1 h. DCs were stained for 1 h with anti-CD11c-AF488 (hamster anti-mouse, clone N418; 1:100), and nuclei were detected with DAPI. For the staining of gp38 + FRC networks and CCL21, slides were blocked for 30 min with 10% goat serum. Slides were then incubated for 1.5 h at room temperature with a hamster anti-mouse gp38 and a rabbit anti-mouse CCL21 antibody, followed by staining with their secondary detection antibodies goat anti-rabbit Alexa Fluor 488 or goat anti-hamster Alexa Fluor 568 in a sequential manner [14] . FDCs were detected with a biotin-coupled rat anti-mouse CD21/CD35 antibody (Biolegend) and with streptavidin Alexa Fluor 488. Immunofluorescence image acquisition of histologies Fluorescently labelled tissue sections were analysed on a Zeiss Axio Imager M2m microscope, equipped with an Apo Tome 2.0 (Carl Zeiss). Images were obtained with a 40 × Plan-Apochromat NA 0.9 objective, or a 20 × Plan-Apochromat NA 0.8 objective. Digital images were processed with the Axio Vision 4.8.2 software (Carl Zeiss) and Adobe Photoshop applying the crop function. Confocal microscopy images were acquired on an upright Leica TCS SPE confocal set-up equipped with a 4-line laser (405/488/532/635 nm) and a continuously variable spectral detector with a bandwidth of 430–750 nm. Digital images were obtained using a × 40 phase contrast plan-apochromat oil objective NA 1.15, DIC WD 0.27 mm. For all acquisition settings, the main beam splitter was 405/532, 488/633 nm. Serial z-stacks were obtained at 0.9 μm intervals. Images were processed using the Leica LAS AF software (Leica) and Adobe Photoshop applying the crop function. RNA isolation, reverse transcription and RT–qPCR DCs from naive B6 mice or recipient mice 10 or 13 days after E μ -Myc lymphoma cell transfer were isolated with collagenase D digestion of spleen (Roche; 2 mg ml −1 in RPMI/2% FCS, 30 min, 37 °C) under frequent agitation. Reaction was stopped with RPMI/5 mM EDTA (final concentration). DCs were positively selected using magnetic sorting with a CD11c MACS bead kit (Miltenyi). Then, cells were further purified using FACS sorting, employing CD11c + and I-A b+ immunostaining. Purity of DCs was usually greater >98% (see Supplementary Fig. S3a ). Total RNA of DCs (1 × 10 6 ) was extracted using the RNeasy Mini Kit (Qiagen). RNA (700 ng) was transcribed into cDNA employing the RT [2] First Strand Kit (SA Biosciences). Gene arrays used were the Mouse Cancer Pathway Finder, Signal Transduction Pathway Finder and Inflammatory Response and Autoimmunity Array (all from SA Biosciences). Each array exhibits 84 different genes. For PCR array data analysis the iQ 5 Optical System software (Bio-Rad) was used. This algorithm performs all ΔΔ C t based fold-change calculations of the gene of interest normalized to the relative quantities of the reference genes Actin beta, GAPDH, Hsp90, Hprt1 and Gusb . For the detection of IGF-1 gene expression, a TaqMan-based qRT–PCR gene expression assay was used (Applied Biosystems). Briefly, DCs from naive Wt (B6), lymphoma-challenged Wt or C/EBPβ −/− mice were recovered using MACS and FACS sorting. Total RNA was extracted using the RNeasy Micro Kit (Qiagen) and further processed as described [68] . The primer sets for GAPDH and IGF-1 and PCR conditions were as predefined by the manufacturer (Applied Biosystems). Antigen-specific T-cell proliferation assay in vivo CD4 + spleen cells from OT-II transgenic mice were purified by negative selection applying magnetic cell sorting as to the manufacturer's instructions (MACS; Miltenyi Biotec). Usually, purity of isolated naive transgenic T cells was in the range of 90%. Cells were labelled with the fluorescent dye eFluor670 before adoptive transfer into naive (non-tumour-challenged) or E μ -Myc lymphoma B-cell-challenged mice (i.v. ), 7–9 days after tumour cell inoculation (i.v.). Twenty hours after T-cell transfer (6–8 × 10 5 cells), mice were immunized s.c. with OVA protein (Sigma-Aldrich; 100 μg) and CpG-ODN 1668 (BioTez Berlin; 25 μg). To determine the proliferation of adoptively transferred T cells, inguinal lymph node cells were prepared, and cells were stained with anticlonotypic T-cell antigen receptor antibody (OT-II) and anti-CD4 antibodies. eFluor 670 dilution was determined with flow cytometry using a FACSCanto II cytometer with FACSDiva and the FloJo software. To gate only the proliferative fraction, in each assay naive or tumour-challenged mice were left non-immunized. Cytometric bead array Serum levels and tissue culture supernatants containing IL-6, IL-10, IFN-γ, TNF-α, MCP-1/CCL2 and IL-12p70 were measured using the Cytometric Bead Array Mouse Inflammation Kit (BD Biosciences) according to the manufacturer’s instructions. Cytokine concentrations were indicated by the mean fluorescent intensity and calculated using standard curves and the FCAP Array v1.0.1 software. Detection of cytokines by ELISA For the determination of IGF-1 in tissue culture supernatants, a Quantikine Mouse IGF-1 ELISA kit (R&D Systems) was employed exactly as recommended by the manufacturer. DCs from lymphoma-bearing mice were recovered by collagenase treatment, followed by CD11c-bead-mediated MACS separation (Miltenyi). DCs were cultured for 4 h in RPMI 1640 containing 5% FCS and in the presence of PMA and ionomycin. Determination of IGF-1 content in cell-free culture supernatant was carried out in the same manner as before. Fort the determination of HGF, primary E μ -Myc lymphoma B cells at a purity of >90% were obtained from diseased animals and cultured in lymphoma medium as detailed before. Cells were stimulated with PMA and ionomycin, and cell-free culture supernatant was analysed after 4 h with a HGF ELISA kit (RayBiotech) exactly as recommended by the manufacturer. Western blot analysis DCs from naive B6 mice or lymphoma-challenged animals (days 7–10 after i.v. injection) were generated by collagenase treatment of the spleen, followed by MACS and FACS sorting as shown before. To detect C/EBPβ, whole-cell lysates were prepared in 8 M urea/50 mM Tris–HCl (pH 7.5) lysis buffer. Samples were sonicated, and protein was quantitated with the Bradford assay. Proteins were analysed with western blot analysis and probed with a polyclonal rabbit anti-C/EBPβ antibody (1:250; Santa Cruz, sc-150). To normalize protein amounts, blots were probed for GAPDH expression. Proteins were visualized by chemiluminescence (ECL kit; Thermo Scientific). Densitometric quantification of gel bands was performed using the Image J software. The ratio between the long LAP/LAP* and the short LIP isoform was then calculated and expressed in a bar graph. Statistical analysis Results are expressed as the arithmetic means±s.d. or as arithmetic means±s.e.m., as indicated. Values of P <0.05 were considered statistically significant, as determined by the unpaired Mann–Whitney test for non-normally distributed data, or the two-tailed unpaired Student’s t -test for normally distributed data, where appropriate. How to cite this article: Rehm, A. et al . Dendritic cell-mediated survival signals in Eμ- Myc B-cell lymphoma depend on the transcription factor C/EBPβ. Nat. Commun. 5:5057 doi: 10.1038/ncomms6057 (2014).